Rational design of a chalcogenopyrylium-based surface-enhanced resonance Raman scattering nanoprobe with attomolar sensitivity High sensitivity and specificity are two desirable features in biomedical imaging. Raman imaging has surfaced as a promising optical modality that offers both. Here we report the design and synthesis of a group of near-infrared absorbing 2-thienyl-substituted chalcogenopyrylium dyes tailored to have high affinity for gold. When adsorbed onto gold nanoparticles, these dyes produce biocompatible SERRS nanoprobes with attomolar limits of detection amenable to ultrasensitive in vivo multiplexed tumour and disease marker detection. Surface-enhanced Raman scattering (SERS) is rapidly gaining interest in the field of biomedical imaging [1] , [2] , [3] . By adsorbing a molecule on a noble metal surface, the weak Raman scattering of a molecule (only 1 in ~10 7 photons induces Raman scattering) is massively amplified (enhancement factor 10 7 −10 10 ) [4] , [5] , [6] . This phenomenon creates a spectroscopic technique that not only has high sensitivity (10 −9 –10 −12 M limits of detectability), but also the potential for multiplexing capabilities due to the unique vibrational structure of adsorbed molecules [7] , [8] , [9] . These characteristics have prompted the use of SERS in a wide array of biomedical imaging applications [2] , [10] , [11] , [12] , [13] , [14] , [15] , [16] , [17] . Orders-of-magnitude higher sensitivities (10 −12 –10 −14 M) can be achieved utilizing Raman reporters that are in resonance with the incident laser, thereby producing surface-enhanced resonance Raman scattering (SERRS) nanoprobes [18] , [19] , [20] . Absorption of light by biological tissue is minimal in the near-infrared (NIR) window and, as a consequence, most optical biomedical applications use NIR detection lasers. While a great deal of attention has been given to dye molecules that absorb light in the visible region, less work has been devoted to developing Raman reporters with absorption maxima that are resonant with NIR detection lasers. The most common Raman reporters are members of the cyanine class of dyes [21] . Herein we report thiophene-substituted chalcogenopyrylium (CP) dyes as a new class of ultra bright, NIR-absorbing Raman reporters. One notable feature of the pyrylium dyes is the ease in which a broad range of absorptivities can be accessed, and consequently be matched with the NIR light source by careful tuning of the dye’s optical properties. Specifically, the large differences in absorption maxima introduced by switching the chalcogen atom is a useful property of this dye class [22] . Another important consideration is the affinity of the reporter for the surface of gold. Since the SERS effect decreases exponentially as a function of distance from the nanoparticle [23] , it is important that the Raman reporter is near the gold surface. The 2-thienyl substituent provides a novel attachment point to gold for Raman reporters. The 2-thienyl group is not only part of the dye chromophore, but also can be rigorously coplanar with the rest of the chromophore [24] . This allows the dye molecules to be in close proximity to the nanoparticle surface, creating a brighter SERRS signal. Chalcogenopyrylium dye synthesis and characterization Cationic CP dyes 1 – 3 , with absorption maxima near the 785-nm emission of the detection laser were synthesized as outlined in Fig. 1a . The addition of MeMgBr to the known chalcogenopyranones [25] ( 4 , 6 ), followed by dehydration with the appropriate acid (HZ), yields 4-methyl pyrylium compounds ( 5 , 7 ) with the desired counterion (PF 6 − or ClO 4 − ) [22] , [26] , [27] . The condensation of 7 with N , N -dimethylthioformamide in Ac 2 O, and subsequent hydrolysis of the intermediate iminium salt yields the (chalcogenopyranylidene)acetaldehyde 8 , the penultimate compound leading to trimethine CP dyes [22] . Condensation of 4-methylpyrylium salt 5 and the (chalcogenopyranylidene)acetaldehyde 8 bearing the desired R groups and chalcogen atom in hot Ac 2 O (ref. 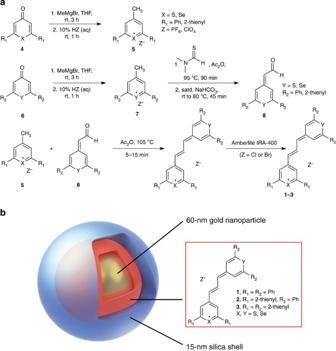Figure 1: Synthesis and structure of the SERRS reporters and SERRS nanoprobe. (a) Reaction scheme for the synthesis of pyrylium-based SERRS reporters (1−3). (b) A 60-nm gold core (yellow) encapsulated in a 15-nm thick chalcogenopyrylium dye (red; Ph, phenyl)-containing silica shell (blue). The structure, yields and optical properties of the different chalcogenopyrylium-based Raman reporters are shown in the table. 26 ) forms the final dye compounds 1 − 3 that are substituted with 2-phenyl or 2-thienyl groups, and different combinations of chalcogen atoms (S or Se) ( Table 1 ). The Cl − and Br − counterions of dye 1a were accessed by treating the PF 6 − salts with an Amberlite ion exchange resin. Figure 1: Synthesis and structure of the SERRS reporters and SERRS nanoprobe. ( a ) Reaction scheme for the synthesis of pyrylium-based SERRS reporters ( 1 − 3 ). ( b ) A 60-nm gold core (yellow) encapsulated in a 15-nm thick chalcogenopyrylium dye (red; Ph, phenyl)-containing silica shell (blue). The structure, yields and optical properties of the different chalcogenopyrylium-based Raman reporters are shown in the table. Full size image Table 1 Chalcogenopyrylium dye structural and optical characteristics. Full size table SERRS nanoprobe synthesis and characterization CP dyes 1 − 3 were dissolved in dry N , N -dimethylformamide (DMF), at a concentration between 1.0 and 10 mM, and were subsequently used to generate the SERRS nanoprobes. The SERRS nanoprobes consist of a gold core onto which the SERRS reporter is adsorbed, which is then protected by an encapsulating silica layer ( Fig. 1b , Table 1 ). The pyrylium-based SERRS nanoprobes were synthesized by encapsulating 60-nm spherical citrate-capped gold nanoparticles via a modified Stöber procedure [28] , [29] , [30] in the presence of the reporter. After 25 min, the reaction was quenched by the addition of ethanol and the SERRS nanoprobes were collected through centrifugation. Typically, the as-synthesized SERRS nanoprobes had a mean diameter of ~100 nm (non-aggregated; Supplementary Figs 1 and 2 ). Effect of counterion on colloidal stability and SERRS signal In previous reports, the dye counterion was shown to affect the structural and electronic properties of polymethine dyes [31] and the solubility of CP dyes [32] . Since SERRS is highly dependent on these factors, we evaluated the effect of the counterion (Z − ) on the SERRS spectrum, intensity and colloidal stability of the pyrylium-based SERRS nanoprobes. We compared chloride (Cl − ), bromide (Br − ), perchlorate (ClO 4 − ) and hexafluorophosphate (PF 6 − ) as counterions for CP dye 1a . The SERRS nanoprobes were synthesized in the presence of equimolar amounts (10 μM) of CP dye 1a ·Z − (where Z − =Cl − , Br − , ClO 4 − or PF 6 − ). The counterion introduces almost no difference in optical properties such as absorption maxima and extinction coefficient. Furthermore, with the exception of the chloride counterion, the Raman shifts and intensity of 1a were minimally affected by the different counterions ( Fig. 2a ). The colloidal stability, however, was shown to be highly counterion dependent ( Fig. 2b , Supplementary Fig. 1 and Supplementary Table 1 ). The least chaotropic counterion, Cl − , strongly destabilized the gold colloids and caused aggregation of SERRS nanoprobes utilizing 1a as a reporter as evidenced by the strong absorption between 700 and 900 nm. The strongest chaotropic anion, PF 6 − , did not affect colloidal stability during the synthesis of SERRS nanoprobes as evidenced by the strong absorption at 540 nm and low absorbance between 700 and 900 nm (monomeric 60-nm spherical gold nanoparticles have an absorption maximum around 540 nm). Since the PF 6 − anion induced the least nanoparticle aggregation, it was used for further SERRS experiments. 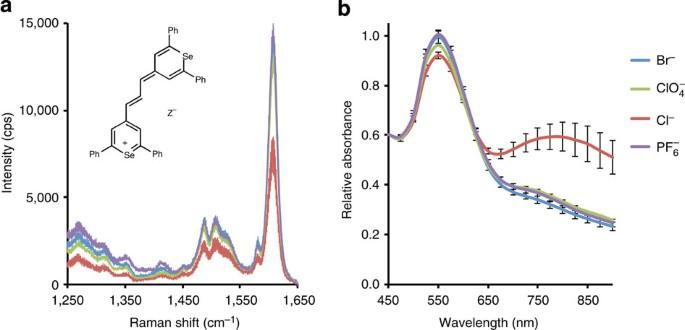Figure 2: The effect of the counterion on colloidal stability. (a) The effect of the counterion (Z−) on SERRS intensity (785 nm, 50 μW, 1.0 s acquisition time, 5 × objective). Inset: Structure of CP dye1a(Ph, phenyl). (b) Effect of counterion on the colloidal stability of CP-dye1a-based SERRS nanoprobes (n=3, error bars represent s.d.; See alsoSupplementary Fig. 1;Supplementary Table 1). Figure 2: The effect of the counterion on colloidal stability. ( a ) The effect of the counterion (Z − ) on SERRS intensity (785 nm, 50 μW, 1.0 s acquisition time, 5 × objective). Inset: Structure of CP dye 1a (Ph, phenyl). ( b ) Effect of counterion on the colloidal stability of CP-dye 1a -based SERRS nanoprobes ( n =3, error bars represent s.d. ; See also Supplementary Fig. 1 ; Supplementary Table 1 ). Full size image Effect of increased affinity on colloidal stability and SERRS signal We also examined the SERRS signal intensity as a function of the number of sulphur atoms in the dye. Sulphur-containing functionality has been used frequently to adhere molecules to gold [33] , with several reports using thiol or lipoic acid functional groups to add sulphur-containing functionality [21] , [34] . In our structures, 2-thienyl groups attached to the 2- and 6- positions of the dye were used to bind the dyes to the gold surface. We also explored the impact of the chalcogen atoms in the CP core, switching a Se ( 1a and 2a ) to S ( 1b and 2b ). The chalcogen switch was used to increase semicovalent interactions with the gold surface, and also to create a chromophore that had a more resonant absorption with the 785-nm detection laser ( Table 1 ). CP dyes 1 − 3 were used at a final concentration of 1.0 μM, which prevented nanoparticle aggregation for dye 3 . Fig. 3a shows the molecular structures of the CP dyes. The SERRS intensity of the different as-synthesized pyrylium-based SERRS nanoprobes, which were synthesized at equimolar reporter concentrations, were measured at equimolar SERRS nanoprobe concentrations at low laser power to prevent CCD-saturation (50 μW, 1.0 s acquisition time, 5 × objective). We specifically focused on the 1,600 cm −1 peak, which corresponds to aromatic ring stretching modes; and is a mode shared by CP dyes 1 – 3 . The SERRS signal intensity of the 1,600 cm −1 peak increased significantly as the number of 2-thienyl substituents increased ( Fig. 3b , Supplementary Table 1 ) without causing significant aggregation ( Fig. 3c , Supplementary Fig. 2 and Supplementary Table 1 ). Thus, 3 produced the highest SERRS signal, which was significantly more intense than 2a / 2b or 1a / 1b ( P <0.05) and 2a / 2b were significantly more intense than 1a / 1b ( P <0.05). There was a less noticeable, but significant, increase from the chalcogen switch in the core ( 1a / 1b and 2a/2b being significantly different ( P <0.05)). This strongly supports the hypothesis that 2-thienyl groups are an effective means of adhering dyes to gold, resulting in brighter SERRS nanoprobes. 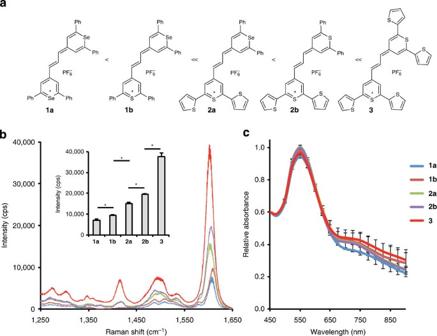Figure 3: The SERRS intensity as a function of dye affinity for the gold surface. (a) Molecular structures of the adsorbed CP dyes (1–3) arranged by increased number of 2-thienyl substituents (Ph, phenyl). (b) SERRS spectra of the CP-based SERRS nanoprobes. The SERRS spectra were baseline corrected to allow proper comparison. (For the non-baseline corrected spectra seeSupplementary Fig. 3). Inset: intensity of the 1,600 cm−1peak (n=3; error bars represent s.d., *P<0.05; an unpaired Student’st-test was performed). (c) Colloidal stability of the CP-based SERRS nanoprobes as determined by LSPR measurements (n=3; error bars represent s.d.; See alsoSupplementary Fig. 2;Supplementary Table 1). Figure 3: The SERRS intensity as a function of dye affinity for the gold surface. ( a ) Molecular structures of the adsorbed CP dyes ( 1 – 3 ) arranged by increased number of 2-thienyl substituents (Ph, phenyl). ( b ) SERRS spectra of the CP-based SERRS nanoprobes. The SERRS spectra were baseline corrected to allow proper comparison. (For the non-baseline corrected spectra see Supplementary Fig. 3 ). Inset: intensity of the 1,600 cm −1 peak ( n =3; error bars represent s.d., * P <0.05; an unpaired Student’s t -test was performed). ( c ) Colloidal stability of the CP-based SERRS nanoprobes as determined by LSPR measurements ( n =3; error bars represent s.d. ; See also Supplementary Fig. 2 ; Supplementary Table 1 ). Full size image Comparison of CP-dye 3 with a cyanine-based SERRS reporter To assess the quality of our optimized nanoprobe, thiopyrylium dye 3 and commercially available IR792 ( Fig. 4a ), which has been previously used to generate surface-enhanced resonance Raman scattering nanoprobes [35] , were studied. A direct comparison of the nanoprobes synthesized in the presence of equimolar (1.0 μM) amounts of 3 and IR792 shows a five- to sixfold higher signal for nanoprobes generated with dye 3 ( Fig. 4b ). It is interesting to note that a fluorescence background is minimal in the SERRS spectra of the CP- and cyanine-based SERRS nanoprobes ( Supplementary Fig. 3 ). Whereas fluorescence interference would not be expected from CP dyes containing heavy chalcogens that enhance intersystem crossing [36] , fluorescence interference could be expected for the cyanine dye IR792 . In fact, when equimolar amounts of the CP dyes 1 − 3 and IR792 were incorporated in silica (without gold nanoparticle), IR792 demonstrated strong fluorescence when excited at 785 nm (50 μW, 1.0 s acquisition time), while minimal fluorescence was observed for CP 1 – 3 . As shown in Fig. 4b and Supplementary Fig. 3 , the fluorescence interference of the cyanine dye IR792 is minimal in its SERRS spectrum. This is due to quenching effects near the surface of the nanoparticle [37] . 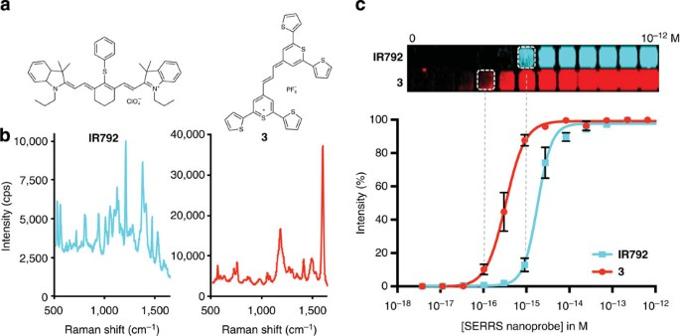Figure 4: Comparison of the SERRS signal intensity of the optimized CP-dye3versus a widely used resonant dye IR792. (a) Structure of the resonant dyeIR792and chalcogenopyrylium dye3. (b) SERRS intensity of an equimolar amount of anIR792-based SERRS nanoprobe and a3-based SERRS nanoprobe that were synthesized with an equimolar amount of the dyes. (c) Limits of detection of theIR792- (cyan) and3- (red) based SERRS nanoprobes were performed in triplicate and determined to be 1.0 fM and 100 aM, respectively (error bars represent s.d.; see alsoSupplementary Fig. 4). Figure 4: Comparison of the SERRS signal intensity of the optimized CP-dye 3 versus a widely used resonant dye IR792. ( a ) Structure of the resonant dye IR792 and chalcogenopyrylium dye 3 . ( b ) SERRS intensity of an equimolar amount of an IR792 -based SERRS nanoprobe and a 3 -based SERRS nanoprobe that were synthesized with an equimolar amount of the dyes. ( c ) Limits of detection of the IR792 - (cyan) and 3 - (red) based SERRS nanoprobes were performed in triplicate and determined to be 1.0 fM and 100 aM, respectively (error bars represent s.d. ; see also Supplementary Fig. 4 ). Full size image A concentration series of the as-synthesized SERRS nanoprobes was generated in triplicate manner ( Supplementary Fig. 4 ) to determine the limit of detection (LOD) of both nanoprobes. Fig. 4c shows the LOD for IR792 -based nanoprobes to be 1.0 fM, while 3 -based nanoprobes had a 10-fold lower LOD, 100 aM. To our knowledge this is the lowest reported LOD utilizing a biologically relevant NIR excitation source. We also evaluated the serum stability of the 3 -based SERRS nanoprobe. The SERRS nanoprobe was shown to be serum stable (no significant difference between t =1 h and t =48 h) for at least 48 h ( Supplementary Fig. 5 ; Supplementary Methods ). This is supported by a study by Thakor et al . [38] who have shown that SERS nanoparticles of similar size and composition remain stable in vivo for >2 weeks. In vivo comparison of EGFR-targeted 3- or IR792-SERRS nanoprobes The ability of our SERRS nanoprobe to delineate tumour tissue in vivo was assessed by utilizing CP dye 3 and IR792 -based SERRS nanoprobes functionalized with an epidermal growth factor receptor (EGFR)-targeting antibody. Equimolar amounts (15 fmol g −1 ) of these two EGFR-targeted nanoprobes were injected intravenously into athymic nude mice that had been inoculated 2 weeks prior with the EGFR-overexpressing cell line A431 (1 × 10 6 cells). After 18 h, the skin around the tumour was carefully peeled back and multiplexed Raman imaging of the tumour site and surrounding tissue was performed ( Figs 5 and 6 ). A Raman map was generated and the signals from the multiplexed SERRS nanoprobes were deconvoluted by applying a direct classical least square algorithm (DCLS) [7] . The SERRS signal from both nanoprobes was more intense for the tumour site than for the surrounding tissue, showing that the EGFR-targeted SERRS nanoprobes had selectively localized at the tumour site. The SERRS signal intensity in the tumour was approximately 3 × higher for the 3 -based SERRS nanoprobe than for the otherwise identical IR792 -based SERRS nanoprobe. Ex vivo multiplexed Raman imaging of the tumour showed Raman signal of the EGFR-targeted SERRS nanoprobes throughout the tumour with the exception of a hypointense Raman region in the centre of the tumour. Hematoxyolin and eosin and immunohistochemical staining for EGFR was performed ( Supplementary Methods ) and revealed that the hypointense Raman region corresponded with an area of necrosis, which explains the lack of SERRS nanoprobe accumulation and decreased Raman signal. In addition, to validate EGFR targeting, we injected A431-tumour-bearing mice with cetuximab (50 pmol g −1 ) 3 h before injection with the EGFR-targeted SERRS nanoprobes. Preblocking of EGFR by cetuximab resulted in decreased accumulation of the EGFR-targeted SERRS nanoprobes within the tumours of animals that were injected with cetuximab before EGFR-targeted SERRS nanoprobe injection as compared with animals that were injected with EGFR-targeted SERRS nanoprobes and were not preinjected with cetuximab ( Supplementary Fig. 6 ). 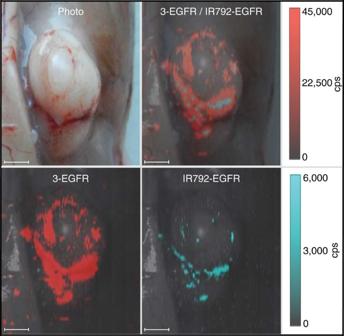Figure 5: Comparison between EGFR-targeted IR792- or 3-based SERRS nanoprobes in an A431 tumour xenograft. Female nude mice (n=5) bearing A431 xenograft tumours were injected intravenously via tail vein with an equimolar amount of EGFR-antibody (cetuximab)-conjugatedIR792- and CP3-based SERRS nanoprobes (15 fmol g−1per probe; total injected dose: 30 fmol g−1). After 18 h, the tumours were imagedin situby Raman (10 mW, 1.5 s acquisition time, 5 × objective). The chalcogenopyrylium dye3-based SERRS nanoprobe (red) provided ~3 × higher signal than theIR792-based SERRS nanoprobe (cyan; 22.442 versus 7.313 cps cm−2, respectively). All scale bars represent 2.0 mm. Figure 5: Comparison between EGFR-targeted IR792- or 3-based SERRS nanoprobes in an A431 tumour xenograft. Female nude mice ( n =5) bearing A431 xenograft tumours were injected intravenously via tail vein with an equimolar amount of EGFR-antibody (cetuximab)-conjugated IR792 - and CP 3 -based SERRS nanoprobes (15 fmol g −1 per probe; total injected dose: 30 fmol g −1 ). After 18 h, the tumours were imaged in situ by Raman (10 mW, 1.5 s acquisition time, 5 × objective). The chalcogenopyrylium dye 3 -based SERRS nanoprobe (red) provided ~3 × higher signal than the IR792 -based SERRS nanoprobe (cyan; 22.442 versus 7.313 cps cm −2 , respectively). All scale bars represent 2.0 mm. 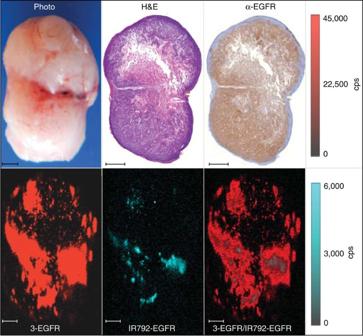Figure 6: Immunohistochemistry andex vivoRaman imaging of the A431 tumour. The excised tumour was scanned by Raman imaging (10 mW, 1.5 s acquisition time, 5 × objective), fixed in 4% paraformaldehyde, and processed for hematoxyolin and eosin staining and anti-EGFR immunohistochemistry. With the exception of a hypointense Raman region in the centre of the tumour, the tumour homogenously expressed EGFR and the EGFR-targeted SERRS nanoprobes had accumulated throughout the tumour. The hypointense Raman area corresponds to a highly necrotic region within the tumour, which explains the lack of SERRS nanoprobe accumulation and decreased Raman signal. All scale bars represent 1.0 mm. Full size image Figure 6: Immunohistochemistry and ex vivo Raman imaging of the A431 tumour. The excised tumour was scanned by Raman imaging (10 mW, 1.5 s acquisition time, 5 × objective), fixed in 4% paraformaldehyde, and processed for hematoxyolin and eosin staining and anti-EGFR immunohistochemistry. With the exception of a hypointense Raman region in the centre of the tumour, the tumour homogenously expressed EGFR and the EGFR-targeted SERRS nanoprobes had accumulated throughout the tumour. The hypointense Raman area corresponds to a highly necrotic region within the tumour, which explains the lack of SERRS nanoprobe accumulation and decreased Raman signal. All scale bars represent 1.0 mm. Full size image Effective biomedical imaging requires low limits of detection and high specificity for biological targets. Raman imaging has surfaced as an optical imaging modality that has the promise to enable both. While the Raman effect is relatively weak (1 in 10 7 photons), the Raman scattering cross-section of a molecule can be massively amplified by noble metal surfaces [4] , [5] , [6] . Here we demonstrated that rational SERRS reporter design afforded SERRS nanoprobes with unprecedented limits of detection: 100 aM. This is, to the best of our knowledge, the lowest reported limit of detection at near-real-time detection (≤2.0 s acquisition times) for SERRS nanoprobes that are compatible with a NIR light source. As a comparison, non-resonant SERS nanoprobes are in the 0.1−1.0 pM range (1,000−10,000-fold less sensitive) [2] , while reported detection limits of SERRS nanoprobes are >17 fM at near-real-time detection [39] . Others have reported a 0.4 fM detection limit; however, this was acquired through cumulative data acquisition with an acquisition time ≥60 s, which is not practical for biomedical imaging applications [35] . We believe the unprecedented limit of detection of our novel SERRS nanoprobe is due to several factors. First, we demonstrate that rational design and optimization of the SERRS reporter is important to achieve efficient ‘loading’ on the nanoparticle. Our results demonstrate that the counterion and gold surface affinity are important considerations. For instance, while the chaotropic PF 6 − anions stabilized the dye–nanoparticle system during silica shell formation in ethanol, the system becomes more destabilized with Cl − (more kosmotropic) ions present. Chloride-induced aggregation of colloidal dispersions in relation to SERS has been studied. Natan and colleagues [40] demonstrated that the strongest enhancements were obtained from aggregates with effective diameters of <200 nm and aggregates with sizes >200 nm did not generate appreciable SERS intensities. The aggregates that were induced by the chloride counterion in our system were >200 nm ( Supplementary Fig. 1 ), which might explain the reduced SERRS signal when chloride is used as a counterion. Others have shown that the kosmotropic chloride ion could induce reorientation of the dye on the surface, which could also contribute to the reduced SERRS intensities [41] . However, while we did observe a decrease in the SERRS signal intensity when chloride is present, we did not find any appreciable differences between the Raman spectra of the dyes when different counterions were used, which would have been expected if the molecule had reoriented on the surface. Since the most chaotropic counterion, PF 6 − , induced the least aggregation and generated robust SERRS signal intensities, we used PF 6 − as a counterion. Next, we showed that an increase in affinity of the SERRS reporter for the gold nanoparticle surface via incorporation of 2-thienyl functional groups considerably increased the SERRS signal without inducing aggregation. Others have reported the functionalization of NIR dyes with thiol or lipoic acid functional groups. In contrast to a 2-thienyl substituent, thiol and lipoic acid functional groups offer no benefit to the optical properties of the dye, and as a tether, do not allow the dye to be as close to the gold surface [34] . Moreover, based on the absorption spectra of reported lipoic acid-modified cyanine dye–gold nanoparticle conjugates, it is clear that lipoic acid-modified dyes promote aggregation [21] . Finally, the strategy chosen to stabilize the SERRS nanoprobe is a key factor. Others have reported using either surfactants or thiolated polymers to stabilize their SERRS nanoparticles [35] , [39] , [42] . However, such stabilizing agents compete with the SERRS reporter for the surface of the nanoparticle, which leads to lower SE(R)RS-signal. We achieved very low limits of detection by using a primerless silication procedure in which the silica not only served as a stabilizing agent, but also as a matrix to contain our optimized CP-based SERRS reporter. Since silica has much lower affinity for the gold than the applied SERRS reporters, attomolar limits of detection were achieved. The CP dyes represent a new class of SERRS reporters. Selection of the right combination of chaotropic counterions and increased affinity of the SERRS reporter for the gold nanoparticle’s surface produces stable SERRS nanoprobes with exceptionally low limits of detection (attomolar range). The low limit of detection (that is, close to single nanoparticle detection) in combination with the high resolution of Raman imaging enables highly sensitive and specific near real-time tumour delineation and, as a result of the fingerprint-like spectra of the different SERRS nanoprobes, can offer multiplexed disease marker detection in vivo . Materials Chalcogenopyrylium dye synthesis and characterization . All reactions were performed open to air. Concentration in vacuo was performed on a rotary evaporator. NMR spectra were recorded at 300 or 500 MHz for 1 H and at 75.5 MHz for 13 C with residual solvent signal as internal standard. If a mixture of CD 2 Cl 2 and CD 3 OD was used to acquire 1 H NMR, the peak for CH 2 Cl 2 was used as the internal standard. UV/VIS-near-IR spectra were recorded in quartz cuvettes with a 1-cm path length. Melting points were determined with a capillary melting point apparatus and are uncorrected. Non-hygroscopic compounds have a purity of ≥95% as determined by elemental analyses for C, H and N. Experimental values of C, H and N are within 0.3% of theoretical values. 13 C NMR was not recorded for pyrylium dyes due to limited solubility in common NMR solvents. Chalcogenopyranones [25] 4 and 6 were made according to literature procedures as were 4-methylchalcogenopyrylium compounds 5 and 7 (refs 22 , 25 , 26 , 27 ). Preparation of 4-(2,6-di(thiophen-2-yl)-4H-thiopyran-4ylidene)acetaldehyde ( 8 , Y=S, R 2 =2-thienyl) . 4-Methyl-2,6-di(thiophen-2-yl)thiopyrylium hexafluorophosphate (0.350 g, 0.833 mmol), N,N -dimethylthioformamide (0.213 ml, 2.50 mmol) and Ac 2 O (3.0 ml) were combined in a small round-bottom flask and heated at 95 °C for 1 h. After cooling to ambient temperature an additional portion of Ac 2 O (2.0 ml) was added and the solution diluted with ether. The formed iminium salt was allowed to precipitate in the freezer overnight, and then isolated by filtration to yield a bright orange solid. This solid was dissolved in CH 3 CN (3.0 ml) and saturated aqueous NaHCO 3 (3.0 ml) was added. This mixture was heated to 80 °C over 15 min, and kept at that temperature for 30 min. After diluting with H 2 O (30 ml) the product was extracted with CH 2 Cl 2 (3 × 50 ml), dried with Na 2 SO 4 and purified on SiO 2 with a 10% EtOAc/CH 2 Cl 2 eluent (R f =0.71) to yield a yellow oil that was recrystallized in CH 2 Cl 2 /hexanes to yield 0.219 g (87%) of a yellow crystalline solid, mp 143–144 °C: 1 H NMR (500 MHz, CDCl 3 ) δ 9.84 (d, 1 H, J =6.0 Hz), 8.26 (s, 1 H), 7.45-7.39 (m, 4 H), 7.13-7.11 (m, 2 H), 6.88 (s, 1 H), 5.72 (d, 1 H, J =6.5 Hz); 13 C NMR (75.5 MHz, CDCl 3 ) δ 188.05, 146.43, 139.36, 139.07, 137.33, 136.65, 128.16, 127.78, 127.58, 126.30, 126.01, 122.48, 117.63, 117.48; HRMS (ESI) m/z 302.9971 (calculated for C 15 H 10 OS 3 +H + : 302.9967). Preparation of 4-(2,6-diphenyl-4H-selenopyran-4ylidene)acetaldehyde ( 8 , Y=Se, R 2 =Ph) . 4-Methyl-2,6-di(phenyl)selenopyrylium hexafluorophosphate (0.200 g, 0.439 mmol), N,N -dimethylthioformamide (0.112 ml, 1.32 mmol) and Ac 2 O (4.0 ml) were added to a round-bottom flask and heated at 95 °C for 90 min. After cooling to room temperature CH 3 CN (4.0 ml) was added and the product precipitated by addition of ether and chilling overnight in the freezer. The iminium salt was isolated by filtration, and hydrolysed by dissolving in CH 3 CN (4.0 ml), adding saturated aqueous NaHCO 3 (4.0 ml) and heating the mixture to 80 °C over a 15 min period. The reaction was maintained at this temperature for 30 min, after which the reaction was diluted with H 2 O (50 ml), the product extracted with CH 2 Cl 2 (3 × 30 ml), dried with MgSO 4 and after concentration purified on SiO 2 with first a CH 2 Cl 2 and then a 10% EtOAc/CH 2 Cl 2 (R f =0.70) eluent to yield 0.122 g (82%) of an orange oil: 1 H NMR (500 MHz, CDCl 3 ) δ 10.11 (d, 1 H, J =10.5 Hz), 8.32 (s, 1 H), 7.62-7.46 (m, 9 H), 7.00 (s, 1 H), 5.88 (d, 1 H, J =11.0 Hz); 13 C NMR (75.5 MHz, CDCl 3 ) δ 188.69, 148.44, 147.01, 146.03, 138.65, 138.40, 129.96, 129.90, 129.14, 126.62, 126.44, 126.37, 126.31, 125.67, 120.57, 120.48; HRMS (ESI) m/z 339.0292 (calculated for C 19 H 14 O 80 Se+H + : 339.0283). Preparation of 4-(3-(2,6-diphenyl-4H-selenopyran-4-ylidene)prop-1-enyl)-2,6-diphenylselenopyrylium ( 1a ) (CAS Registry Number: 51848-65-8) . PF 6 − 4-Methyl-2,6-di(phenyl)selenopyrylium hexafluorophosphate (0.190 g, 0.417 mmol), 4-(2,6-diphenyl-4H-selenopyran-4-ylidene)acetaldehyde (0.155 g, 0.459 mmol) and Ac 2 O (3.0 ml) were combined in a round-bottom flask and heated at 105 °C for 10 min. The reaction was cooled to ambient temperature, precipitated with ether and the collected solid recrystallized from CH 3 CN/ether to yield 0.278 g (86%) of a golden-green solid: 1 H NMR (500 MHz, CD 2 Cl 2 ) δ 8.59 (t, 1 H, J =13.5 Hz), 8.40–7.80 (br s, 4 H), 7.71 (d, 8 H, J =7.0 Hz), 7.63-7.59 (m, 12 H), 6.85 (d, 2 H, J =13.0 Hz); analytically calculated for C 37 H 27 Se 2 ·PF 6 : C, 57.38; H, 3.51; F, 14.72. Found: C, 57.34; H, 3.48; F, 14.76; LRMS (ESI) m/z 631.2 (calculated for C 37 H 27 80 Se 2 : 631.0); λ max (CH 2 Cl 2 )=806 nm, ε=2.5 × 10 5 M −1 cm −1 . ClO 4 − 4-Methyl-2,6-di(phenyl)selenopyrylium perchlorate (50.0 mg, 0.122 mol), 4-(2,6-diphenyl-4H-selenopyran-4-ylidene)acetaldehyde (81.4 mg, 0.241 mmol) and Ac 2 O (2.0 ml) were treated as described for the PF 6 − salt to yield 82.0 mg (90%) of a golden-green solid: 1 H NMR (500 MHz, 1:1 CD 2 Cl 2 :CD 3 OD) δ 8.77 (t, 1 H, J =13.5 Hz), 8.60–7.80 (m, 4 H), 7.71 (d, 8 H, J =7.0 Hz), 7.66–7.54 (m, 12 H), 6.83 (d, 2 H, J =14.0 Hz); analytically calculated for C 37 H 27 Se 2 ·ClO 4 : C, 60.96; H, 3.73. Found: C, 60.69; H, 3.83; λ max (CH 2 Cl 2 )=806 nm, ε =2.5 × 10 5 M −1 cm −1 . Cl − The hexafluorophosphate salt (50 mg) was converted to the chloride salt by treating with Amberlite IRA-400 chloride form (200 mg) in a 1:1 CH 2 Cl 2 :MeOH mixture (3.0 ml). This process was repeated two more times after which the product was dissolved in CH 2 Cl 2 , washed with water, the organic layer dried with Na 2 SO 4 , filtered over Celite and after concentration recrystallized from CH 3 CN/ether to yield a bronze solid: 1 H NMR (500 MHz, 3:1 CD 3 OD:CD 2 Cl 2 ) δ 8.87 (t, 1 H, J =13.0 Hz), 8.40–7.80 (m, 4 H), 7.70 (d, 8 H, J =7.0 Hz), 7.56-7.50 (m, 12 H), 6.84 (d, 2 H, J =13.0 Hz); analytically calculated for C 37 H 27 Se 2 ·Cl·4/3H 2 O: C, 64.50; H, 4.34; Cl, 5.15. Found: C, 64.54; H, 4.42; Cl, 4.98; λ max (CH 2 Cl 2 )=806 nm, ε =2.3 × 10 5 M −1 cm −1 . Br − The hexafluorophosphate salt (50 mg) was converted to the bromide salt by treating with Amberlite IRA-400 bromide form (200 mg) in a 1:1 CH 2 Cl 2 :MeOH mixture (3.0 ml). This process was repeated two more times after which the product was dissolved in CH 2 Cl 2 , washed with water, the organic layer dried with Na 2 SO 4 , filtered over Celite and after concentration recrystallized from CH 3 CN/ether to yield a bronze solid: 1 H NMR (500 MHz, 3:2 CD 2 Cl 2 :CD 3 OD) δ 8.79 (t, 1 H, J =13.5 Hz), 8.40–7.80 (br s, 4 H), 7.71 (d, 8 H, J =7.0 Hz), 7.60–7.54 (m, 12 H), 8.50 (d, 2 H, J =13.0 Hz); analytically calculated for C 37 H 27 Se 2 ·Br·H 2 O: C, 61.09; H, 4.02; Br, 10.98. Found: C, 61.08; H, 3.89; Br, 10.77; λ max (CH 2 Cl 2 )=806 nm, ε =2.3 × 10 5 M −1 cm −1 . Preparation of 4-(3-(2,6-diphenyl-4H-thiopyran-4-ylidene)prop-1-enyl)-2,6-diphenylselenopyrylium hexafluorophosphate ( 1b ) (CAS Registry Number: 79054-92-5) . 4-Methyl-2,6-di(phenyl)thiopyrylium hexafluorophosphate (0.128 g, 0.312 mmol), 4-(2,6-diphenyl-4H-selenopyran-4-ylidene)acetaldehyde (0.157 g, 0.344 mmol) and Ac 2 O (2.0 ml) were combined in a round-bottom flask and heated at 105 °C for 10 min. The reaction was cooled to ambient temperature, CH 3 CN (2.0 ml) was added and ether was used to precipitate product from solution to yield 0.196 g (86%) of a copper–bronze solid: 1 H NMR (500 MHz, CD 2 Cl 2 ) δ 8.54 (t, 1 H, J =13.0 Hz), 8.20-7.80 (br s, 4 H), 7.78 (d, 4 H, J =8.0 Hz), 7.70 (d, 4 H, J =7.5 Hz), 7.66–7.58 (m, 12 H), 6.78 (d, 2 H, J =13.5 Hz); analytically calculated for C 39 H 34 O 3 Se 2 ·PF 6 : C, 61.08; H, 3.74. Found: C, 61.10; H, 3.68; LRMS (ESI) m/z 583.3 (calculated for C 37 H 27 S 80 Se: 583.1); λ max (CH 2 Cl 2 )=784 nm, ε =2.0 × 10 5 M −1 cm −1 . Preparation of 4-(3-(2,6-dithiophen-2-yl-4H-thiopyran-4-ylidene)prop-1-enyl)-2,6-diphenylselenopyrylium ( 2a ). 4-Methyl-2,6-di(phenyl)selenopyrylium hexafluorophosphate (0.102 g, 0.225 mmol), 4-(2,6-(thiophen-2-yl)-4H-thiopyran-4-ylidene)acetaldehyde (75.0 mg, 0.248 mmol) and Ac 2 O (3.0 ml) were combined in a round-bottom flask and heated at 105 °C for 5 min. The reaction was cooled to ambient temperature, precipitated with ether and the collected solid recrystallized from CH 3 CN/ether to yield 0.145 g (87%) of a bronze solid, mp 229–231 °C: 1 H NMR [500 MHz, CD 2 Cl 2 ] δ 8.46 (t, 1 H, J =13.0 Hz), 7.71–7.58 (m, 18 H), 7.26 (t, 2 H, J =4.0 Hz), 6.77 (d, 1 H, J =13.0 Hz), 6.70 (d, 1 H, J =14.0 Hz); analytically calculated for C 33 H 23 S 3 Se·PF 6 : C, 53.59; H, 3.13; F, 15.41. Found: C, 53.79; H, 3.13; F, 15.19; HRMS (ESI) m/z 595.0125(calculated for C 33 H 23 S 3 80 Se: 595.0122); λ max (CH 2 Cl 2 )=810 nm, ε =2.5 × 10 5 M −1 cm −1 . Preparation of 4-(3-(2,6-dithiophen-2-yl-4H-thiopyran-4-ylidene)prop-1-enyl)-2,6-diphenylthiopyrylium hexafluorophosphate ( 2b ). 4-Methyl-2,6-diphenylthiopyrylium hexafluorophosphate (30.0 mg, 73.0 μmol), 4-(2,6-(thiophen-2-yl)-4H-thiopyran-4-ylidene)acetaldehyde (24.4 mg, 81.0 μmol) and Ac 2 O (1.0 ml) were combined in a round-bottom flask and heated at 105 °C for 5 min. The reaction was cooled to ambient temperature, CH 3 CN (4.0 ml) was added and ether was used to precipitate product from solution to yield 45.0 mg (88%) of a bronze solid, mp>260 °C: 1 H NMR (500 MHz, CD 2 Cl 2 ) δ 8.44 (t, 1 H, J =13.0 Hz), 8.40–7.80 (br s, 4 H), 7.78 (d, 4 H, J =7.0 Hz), 7.67–7.59 (m, 10 H), 7.24 (t, 2 H, J =4.5 Hz), 6.71 (d, 1 H, J =13.0 Hz), 6.63 (d, 1 H, J =13.5 Hz); analytically calculated for C 33 H 23 S 4 ·PF 6 : C, 57.21; H, 3.35. Found: C, 56.97; H, 3.36; HRMS (ESI) m/z 547.0674 (calculated for C 33 H 23 S 4 : 547.0677); λ max (CH 2 Cl 2 )=789 nm, ε =2.2 × 10 5 M −1 cm −1 . Preparation of 4-(3-(2,6-dithiophen-2-yl-4H-thiopyran-4-ylidene)prop-1-enyl)-(2,6- dithiophen-2-yl)thiopyrylium hexafluorophosphate ( 3 ) (CAS Registry Number: 95410-36-9) . 4-Methyl-2,6-di(thiophen-2-yl)thiopyrylium hexafluorophosphate (11.0 mg, 26.2 μmol), 4-(2,6-(thiophen-2-yl)-4H-thiopyran-4-ylidene)acetaldehyde (9.5 mg, 31.4 μmol) and Ac 2 O (1.0 ml) were combined in a round-bottom flask and heated at 105 °C for 5 min. The reaction was cooled to ambient temperature, CH 2 Cl 2 (2.0 ml) was added and ether was used to precipitate product from solution to yield 17.8 mg (94%) of a bronze solid, mp>260 °C: 1 H NMR (500 MHz, CD 3 CN) δ 8.32 (t, 1 H, J =13.5 Hz), 7.68 (d, 2 H, J =4 Hz), 7.56 (br. s, 4 H) 7.14 (t, 4 H, J =4.5 Hz), 6.48 (d, 2 H, J =13.0 Hz); analytically calculated for C 29 H 19 S 6 ·PF 6 : C, 49.42; H, 2.72. Found: C, 49.19; H, 2.79; HRMS (ESI) m/z 558.9805 (calculated for C 29 H 19 S 6 : 558.9806); λ max (CH 2 Cl 2 )=813 nm, ε =2.8 × 10 5 M −1 cm −1 . Spectral data agree with published spectra [43] . SERRS nanoprobe synthesis Gold nanoparticles were synthesized by adding 7.5 ml 1% (w/v) sodium citrate to 1.0 l boiling 0.25 mM HAuCl 4 . The as-synthesized gold nanoparticles were concentrated by centrifugation (10 min, 7,500 × g , 4 °C) and dialysed overnight (3.5 kDa MWCO; 5 l 18.2 MΩ cm). The dialysed gold nanoparticles (100 μl; 2.0 nM) were added to 1,000 μl absolute ethanol in the presence of 30 μl 99.999% tetraethyl orthosilicate (Sigma Aldrich), 15 μl 28% (v/v) ammonium hydroxide (Sigma Aldrich) and 1 μl CP dye (1−10 mM) in DMF. After shaking (375 rpm) for 25 min at ambient conditions in a plastic container, the SERRS nanoprobes were collected by centrifugation, washed with ethanol and redispersed in water to yield 2.0 nM SERRS nanoprobes. SERRS nanoprobe characterization The as-synthesized SERRS nanoprobes were characterized by transmission electron microscopy (TEM; JEOL 1200ex-II, 80 kV, 150,000 × magnification) to study the SERRS nanoprobe structural morphology. The size and concentration of the SERRS nanoprobes were determined on a Nanoparticle Tracking Analyzer (Malvern Instruments, Malvern, UK). Absorption spectra to determine possible nanoparticle aggregation (typically detectable at wavelengths>600 nm) were measured on an M1000Pro spectrophotometer (Tecan Systems Inc., San Jose, CA). Finally Raman spectra were acquired on a Renishaw InVIA system equipped with a 785-nm laser (Renishaw Inc., Hoffman Estates, IL). All measurements were performed at a laser power of 50 μW (1.0 s acquisition time, 5 × objective). SERRS nanoprobe limit of detection SERRS nanoprobes were synthesized as described above in the presence of an equimolar (1.0 μM) amount of 3 or IR792 . SERRS imaging to determine the limit of detection was performed at 100 mW (2.0 s acquisition time (StreamLine), 5 × objective) on a phantom that consisted of a serially diluted IR792 - or CP dye 3 -based SERRS nanoprobe redispersed in 10 μl water (concentration range 3,000−0.003 fM; n =3). The Raman maps were generated using WiRE 3.4 software (Renishaw) by applying a DCLS algorithm. The Raman images were analysed with ImageJ software and plotted in GraphPad Prism (GraphPad Software Inc., La Jolla, CA). Animal studies All animal experiments were approved by the Institutional Animal Care and Use Committees of Memorial Sloan Kettering Cancer Center. In vivo comparison of EGFR-targeted 3- or IR792-SERRS nanoprobes Eight-to-ten week-old female athymic nude mice ( n =5; Hsd:Athymic Nude -Foxn1 nu ; Harlan Laboratories) were subcutaneously inoculated with the EGFR-overexpressing cell line A431 (1 × 10 6 cells; ATCC CRL-1555). After 2 weeks, the mice were injected with an equimolar amount (15 fmol g −1 ) of EGFR-targeted IR792 - and 3 -based SERRS nanoprobes. The EGFR-targeted SERRS nanoprobes were synthesized as described above in the presence of an equimolar (1.0 μM) amount of 3 or IR792 . The as-synthesized SERRS nanoprobes were subsequently functionalized with sulfhydryl groups by heating the SERRS nanoprobes in 5 ml 2% (v/v) mercaptotrimethoxysilane in ethanol at 70 °C for 2 h. The sulfhydryl-functionalized SERRS nanoprobes were washed with water, redispersed in 10 mM MES buffer (pH 7.1), and conjugated to an EGFR-targeting antibody (cetuximab; Genentech, South San Francisco, CA) with a 4,000 Da heterobifunctional maleimide/ N -hydroxysuccinimide polyethylene glycol linker [44] . Eighteen hours later, the mice were sacrificed by CO 2 asphyxiation. The tumour was exposed and scanned by Raman imaging (10 mW, 1.5 s acquisition time (StreamLine), 5 × objective). The Raman maps were generated using WiRE 3.4 software (Renishaw) by applying a DCLS algorithm. How to cite this article: Harmsen, S. et al . Rational design of a chalcogenopyrylium-based surface-enhanced resonance Raman scattering-nanoprobe with attomolar sensitivity. Nat. Commun . 6:6570 doi: 10.1038/ncomms7570 (2015).